Sauropod dinosaur osteoderms from the Late Cretaceous of Madagascar Osteoderms are bones embedded within the dermis, and are common to select members of most major tetrapod lineages. The largest known animals that bear osteoderms are members of Titanosauria, a diverse clade of sauropod dinosaurs. Here we report on two titanosaur osteoderms recovered from the Upper Cretaceous Maevarano Formation of Madagascar. Each osteoderm was discovered in association with a partial skeleton representing a distinct ontogenetic stage of the titanosaur Rapetosaurus krausei . Combined, these specimens provide novel insights into the arrangement and function of titanosaur osteoderms. Taphonomic data confirm that Rapetosaurus developed only limited numbers of osteoderms in its integument. The adult-sized osteoderm is the most massive integumentary skeletal element yet discovered, with an estimated volume of 9.63 litres. Uniquely, this specimen possesses an internal cavity equivalent to more than half its total volume. Large, hollow osteoderms may have functioned as mineral stores in fecund, rapidly growing titanosaurs inhabiting stressed environments. Osteoderms are widely distributed among archosaurs including crocodylomorphs, aetosaurs and dinosaurs [1] , [2] , [3] , [4] , [5] , [6] . Among dinosaurs, osteoderms are best known from the ornithischian clades Ankylosauria [7] and Stegosauria [8] , [9] , where they develop into a variety of plate- and spine-shaped elements and have a characteristic paramedian distribution as multiple rows enveloping the dorsolateral body surface. Among saurischians, osteoderms have been reported for a single carnivorous dinosaur, the ceratosaurian Ceratosaurus [10] , and a number of titanosaurian sauropods [4] , [5] , [6] . Titanosauria is a diverse clade of sauropods that attained a global distribution by the end of the Cretaceous Period, and includes both the largest terrestrial vertebrates yet known and small-bodied dwarfs [6] . Titanosaurs are the only sauropods known to possess osteoderms, although specific details of the taxonomic identity, anatomical distribution, evolution, and potential function(s) of these elements remain a mystery [4] . Here we report on two recently recovered osteoderms that represent different stages of skeletal ontogeny ( Fig. 1 ). Significantly, these elements reveal that the enormous size of at least some adult Rapetosaurus osteoderms is accompanied by the presence of a large, hollow cavity ( Figs 1h , 2 ). 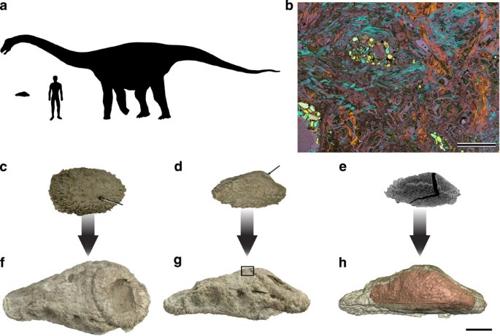Figure 1:Rapetosaurus krauseiosteoderm morphology at two different ontogenetic stages. (a) Silhouette drawings of an adultRapetosaurus krauseiosteoderm (FMNH PR 2342), a 1.8-m-tall human, and an adult specimen ofRapetosaurus krausei, highlighting the large size of the osteoderm. (b) Bone histology of the adult osteoderm ofRapetosaurus krausei, showing densely remodelled, intersecting spicules of fibrolamellar bone and internal resorption cavities and 0.5 cm scale bar. Location of thin section is indicated by the box ing. (c–e) Osteoderm pertaining to a juvenile specimen ofRapetosaurus krausei(UA 9331) with 5 cm scale bar inc, external;d, lateral,e, CT-generated slice illustrating the highly vascularized internal anatomy of this osteoderm. A 2D projection of the twisting sinus that passes through the osteoderm is shown in black. Arrows incanddindicate one exit of this sinus. (f–h) Adult osteoderm ofRapetosaurus krauseiwith 10 cm scale bar inf, external view, depression at right is result of damage during excavation and is not a primary anatomical characteristic. (g) Lateral view with box showing location of histological section shown inb, andh, isometric CT reconstruction with exterior bone rendered transparent and internal cavity (volume=4.88 litres) shown in pink. Wide arrows betweenc–eandf,gindicate the possible ontogenetic development ofRapetosaurusosteoderms. The total volume of the adult osteoderm is 9.63 l. Figure 1: Rapetosaurus krausei osteoderm morphology at two different ontogenetic stages. ( a ) Silhouette drawings of an adult Rapetosaurus krausei osteoderm (FMNH PR 2342), a 1.8-m-tall human, and an adult specimen of Rapetosaurus krausei , highlighting the large size of the osteoderm. ( b ) Bone histology of the adult osteoderm of Rapetosaurus krausei , showing densely remodelled, intersecting spicules of fibrolamellar bone and internal resorption cavities and 0.5 cm scale bar. Location of thin section is indicated by the box in g . ( c – e ) Osteoderm pertaining to a juvenile specimen of Rapetosaurus krausei (UA 9331) with 5 cm scale bar in c , external; d , lateral, e , CT-generated slice illustrating the highly vascularized internal anatomy of this osteoderm. A 2D projection of the twisting sinus that passes through the osteoderm is shown in black. Arrows in c and d indicate one exit of this sinus. ( f – h ) Adult osteoderm of Rapetosaurus krausei with 10 cm scale bar in f , external view, depression at right is result of damage during excavation and is not a primary anatomical characteristic. ( g ) Lateral view with box showing location of histological section shown in b , and h , isometric CT reconstruction with exterior bone rendered transparent and internal cavity (volume=4.88 litres) shown in pink. Wide arrows between c – e and f , g indicate the possible ontogenetic development of Rapetosaurus osteoderms. 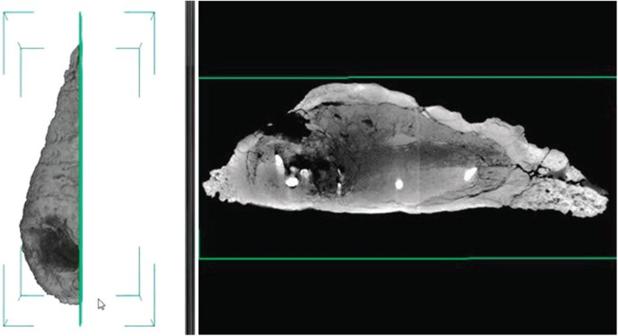Figure 2: CT-scan image of an adultRapetosaurus krauseiosteoderm. The CT scan shows the internal void in FMNH PR 2342, an adultRapetosaurus krauseiosteoderm. The void is filled with unconsolidated sediment. Radio-opaque internal bright spots are secondary deposits of barite (common in Maevarano Formation fossils). The cavity is∼4.9 litres in volume, with the thickness of bone surrounding the external cavity ranging from 1.2 to 3.5 cm. The total volume of the adult osteoderm is 9.63 l. Full size image Figure 2: CT-scan image of an adult Rapetosaurus krausei osteoderm. The CT scan shows the internal void in FMNH PR 2342, an adult Rapetosaurus krausei osteoderm. The void is filled with unconsolidated sediment. Radio-opaque internal bright spots are secondary deposits of barite (common in Maevarano Formation fossils). The cavity is ∼ 4.9 litres in volume, with the thickness of bone surrounding the external cavity ranging from 1.2 to 3.5 cm. Full size image Location The new osteoderms were recovered from locality MAD 93-18 in the Anembalemba Member of the Maevarano Formation (Maastrichtian) [11] . MAD 93-18 includes at least three bone-bearing horizons that yield well-preserved skeletal remains of Rapetosaurus [6] , [12] . Juvenile Rapetosaurus osteoderm anatomy UA (Université d'Antananrivo) 9331, the smallest osteoderm, was collected in association with the caudal vertebrae of a partially articulated skeleton of a juvenile Rapetosaurus (femur length= ∼ 75 cm) in the uppermost bonebed of MAD 93-18. UA 9331 is an ellipsoid osteoderm that measures 14.4cm × 9.2cm × 6.9 cm. Except for a low-relief, relatively smooth midpoint convexity, the majority of the external bone texture of UA 9331 is rugose, characterized by thin, disorganized and densely packed mineralized fibres ( Fig. 1c–e ). Computed tomographic (CT) scans demonstrate that the pristinely preserved outer cortex of dense, compact bone is underlain by a cancellous core of bony trabeculae similar to that of other amniote osteoderms [1] , [2] , [3] , [4] ( Fig. 1e ). Of particular note is a prominent canal that passes uninterrupted through the element ( Fig. 1c–e ). As evidenced by CT scans, this canal widens to form a cavity midway into the osteoderm, within the otherwise cancellous core of the element ( Fig. 1e ). A distinct radiopaque layer of compact bone lines this cavity. CT scans also reveal a horizon of radiopaque compact bone deep within the cancellous core that spans the long axis of the element and intersects with the cavity ( Fig. 1e ). Adult Rapetosaurus osteoderm anatomy FMNH PR (Field Museum of Natural History) 2342, the large osteoderm, was recovered in close association with right and left ischia of an adult-sized Rapetosaurus skeleton (femur length=146 cm) in the basal bonebed of MAD 93-18. This osteoderm measures 57.2 cm × 26.7 cm × 19.2 cm in maximum dimensions and has an estimated volume of 9.63 l, making it the most massive osteoderm ever discovered ( Figs 1a,b,f–h and 2 ). Overall, it resembles an ellipsoid and exhibits the bulb and root morphology noted for some other titanosaur osteoderms [4] . A large ovoid depression on the external surface of the osteoderm reflects damage to the relatively smooth, flat, circular bulb during collection, and is not a primary anatomical characteristic ( Fig. 1f ). The deep surface is characterized by an orthogonal or cross-hatched texture of mineralized fibres punctuated by numerous foramina, whereas the superficial surfaces are relatively smooth and more sparsely vascularized. CT scans ( Fig. 1h ) and exploratory cores ( Fig. 1b ) taken for histological purposes reveal that FMNH PR 2342 is hollow. The void is filled with unconsolidated sediment and contains no broken internal trabeculae. This cavity is ∼ 4.9 l in volume, representing more than 50% of the total volume of the osteoderm. The thickness of bone surrounding this inner cavity varies from 1.2 to 3.5 cm ( Fig. 1f,h ). The inner bony margin of the cavity shows resorptive lacunae consistent with osteoclastic resorption [13] , [14] , [15] and grades into heavily remodelled fibrolamellar bone ( Fig. 1b ). These two specimens represent examples of both juvenile and adult Rapetosaurus osteoderm development. The structural organization (compact cortex, cancellous core) and bone histology of the juvenile specimen (UA 9331) are broadly comparable with those of other archosaurs [1] , [2] , [3] , [4] , [7] . In contrast, the gross anatomical and microscopic structure of the adult-sized specimen (FMNH PR 2342) is unique. The shape and surface texture of Rapetosaurus osteoderms indicates that these elements were low in relief and embedded in the integument as in other vertebrates [1] , [2] , [3] , [14] , [16] . As evidenced from extant taxa, all osteoderms form and reside within the dermis, either adjacent to the interface between the strata superficiale and compactum , or exclusively within the stratum superficiale , and are overlain by the epidermis [1] , [2] , [3] , [14] , [15] , [16] , [17] . The surface texture of Rapetosaurus osteoderms is consistent with the hypothesis that, as in crown group archosaurs, these structures were overlain by epidermal scales [1] , [2] , [3] . The hollow nature of the adult specimen is unique, and we speculate that the juvenile morph remodels to achieve the adult form. We propose that the initially modest vascular sinus present in the juvenile specimen could represent the locus for calcium remobilization and remodelling, resulting in a well-defined hollow rimmed by heavily remodelled bone tissue at the adult stage ( Fig. 1 ). Although osteoderms are a commonly cited feature of titanosaurs, they are relatively rare, with only about 90 specimens known worldwide [4] . Thus, it is not surprising that only 10 osteoderms have been collected among the 141 titanosaur-bearing localities in the Maevarano Formation [5] , [6] , [12] , [18] . Sedimentologic data indicate that recurrent fine-grained debris flows were the predominant burial mechanism for Maevarano Formation vertebrates [11] , [19] , [20] . These viscous debris flows would not have readily entrained and winnowed osteoderms from their respective skeletons, but are predicted to bury them in close proximity to other skeletal remains, as is the case with crocodylomorphs recovered from the same formation [19] . Accordingly, we reason that the integument of Rapetosaurus was not heavily invested with osteoderms. Instead, we hypothesize that Rapetosaurus (and probably most titanosaurs) was characterized by a small number of osteoderms. Furthermore, unlike many osteoderm-bearing archosaurs [1] , [2] , [3] , these elements did not develop pervasively throughout the dermis but were probably restricted to the isolated regions of the integument. Whereas previous descriptions had reported the presence of articulating mosaics of osteoderms from the Maevarano formation [5] , we reinterpret these 'mosaics' as the fragmentary remains of individual adult-sized cavitied elements that were crushed post-mortem. To date, at least four Maevarano Formation osteoderm occurrences consist of these fragmentary remnants of large adult specimens. Although titanosaur phylogeny is currently labile, all published cladograms require multiple independent gains and/or losses of osteoderms [4] , [6] , [21] . This pattern may be genuine, as osteoderms have a sporadic phylogenetic distribution in other clades, with independent evolution of osteoderms at least eight times within Amniota, and at least four times within Archosauria [1] , [2] , [3] . However, in light of the fragile nature of hollow titanosaur osteoderms, some of the perceived losses of osteoderms in titanosaur evolution are more likely attributable to taphonomy. With regard to potential function, osteoderms are often assumed to have a protective role, but this is unlikely for Rapetosaurus osteoderms, because they do not form the imbricated 'armour' observed in other vertebrates [1] , [2] , [3] , [16] , [22] , [23] , [24] . Moreover, protective benefits would seemingly decrease in the vacuous, thin-walled adult structures. Thermoregulatory functions, proposed for osteoderms in crocodylomorphs [1] , [2] , [3] , [22] and squamates [1] , [25] , [26] , are unlikely for Rapetosaurus because its osteoderms are arguably too rare to be effective, especially with their low surface area–volume ratios. The lack of an osteoderm 'pavement' or 'shield' also precludes biomechanical support during locomotion as proposed for crocodyliforms [27] . Display, including mate and species recognition, is probably the most commonly cited explanation for dinosaur osteoderms [7] , [8] , [9] , [10] , but Rapetosaurus osteoderms are nondescript in comparison to the elaborate bony display structures of other dinosaurs [7] , [10] , especially when considered in the context of adult body size [4] , [6] , [12] . Moreover, similarly shaped ellipsoid osteoderms have been attributed to five other titanosaurs on as many continents [4] , reducing the likelihood of a widespread role in species individuation [7] , [9] . Finally, the discovery of several other hollow osteoderms in the Maevarano formation precludes both pathology and individual variation as causes of the internal cavity observed in adult Rapetosaurus . Given the above considerations, we are reluctant to attribute any of the aforementioned functions to the unusual Rapetosaurus osteoderms. Instead, we propose that they might have served as a mineral reservoir. Osteoclastic remodelling of bone mineral is necessary for blood calcium homeostasis [15] , [27] , [28] , [29] and increases seasonally [30] , during oogenesis [23] , and with increased age [13] in extant animals. Osteoderms are often associated with complex vascular networks, including numerous small diameter anastomozing arteries and veins within the stratum superficiale [3] , [14] , [16] , [22] , [25] , [26] , [31] , [32] . These vessels then join larger diameter subcutaneous arterioles and venules [22] , [25] , [26] , [32] . These vascular networks facilitate thermoregulation in some crocodylians [22] and lizards [25] , and also serve as conduits for mobilized mineral reserves from the integument [23] , [25] , [26] , [30] . Like most other sauropods, titanosaurs like Rapetosaurus rapidly attained skeletal maturity [32] and exhibited comparatively high levels of fecundity [33] , both of which place demands on bone mineral reserves [13] , [15] , [22] , [23] , [28] , [29] , [34] , [35] . Moreover, Rapetosaurus inhabited a highly seasonal, semi-arid setting that was characterized by periodic, intense droughts that resulted in recurrent mass mortality [19] , [20] . Only six of the ten other known osteoderm-bearing titanosaurs are derived from well-documented palaeoenvironmental contexts [4] . These taxa also inhabited seasonal, semi-arid to arid palaeoenvironments [36] , [37] , [38] , [39] , [40] , [41] . Under these palaeoenvironmental conditions, we propose that osteoderms may have provided an important, adaptive, integumentary mineral reservoir throughout Rapetosaurus life history (and perhaps in other osteoderm-bearing titanosaurs). In response to physiological demands, calcium and phosphorous were presumably redeployed through osteoclasia and mobilized within a dermal vascular network resulting in the formation of large interior cavities. Under prolonged and/or recurrent stress, it is possible that osteoderms were so extensively remodelled that they became either unrecognizable as distinct elements or too fragile to survive the rigours of burial and fossilization, both of which would account for their rarity in the Maevarano Formation, and the titanosaur record in general. Adult Rapetosaurus bore a few massive, but internally hollow, integumentary skeletal elements. The internal hollow appears to develop through remodelling of the cancellous core observed at juvenile ontogenetic stages, and may have functional implications for mineral storage in fecund, rapidly growing titanosaurs inhabiting stressed environments. Computed tomography CT scanning of FMNH 2342 was done on an NSI M5000 digital real-time and computed tomography system provided by North Star Imaging. A 'Cone-Beam' CT scan was performed acquiring 720 two-dimensional (2D) images during a 360° rotation of the specimen-yielding images at 0.5 degree increments. Resolution of the detector was 2,048×2,048 pixels with magnification of ×1.25 providing an optimum effective three-dimensional (3D) voxel resolution of ∼ 155 microns. The sample was scanned in two halves with maximum penetration power of 450 kV. The smaller specimen was scanned on an NSI M500 digital real-time system with an effective 3D voxel resolution of ∼ 75 microns. The volume of the interior void of FMNH PR 2342 was calculated with software provided by Kinetic Vision via a technique called segmentation, in which pixels are selected either automatically, semi-automatically, or manually on a set of successive 2D images. These 2D images make up a 3D volume when stacked together. Automatic/semi-automatic selection of pixels is based on the iso-value correlating to each pixel of the data set. Once automatic segmentation is complete manual segmentation allowed clean up of areas where noise occurs. The selected pixels are then designated to a material label (for example, exterior surface or interior void). Once the pixels of interest are correctly assigned to a material, then the volume of each material was calculated: FMNH PR 2342 total volume=9,627,075.5 mm 3 ; FMNH PR 2342 interior void volume=4,880,507.5 mm 3 ( Fig. 2 , Supplementary Movie 1 ). Histological analysis Two areas of FMNH PR 2342 were cored with a diamond-coated drill bit perpendicular to the long axis of the element for histological analysis. The first core came from the intersection of the bulb and root ( Fig. 1 ). A second core came from the external surface of the root. Cores were embedded in epoxy resin and mounted to glass slides. Thin-sections were made with an Isomet slow speed diamond saw and hand ground on a lapidary wheel until ∼ 60–80 μm thick. Observations/measurements were made with regular and cross-polarized microscope. Copies of thin-sections are located at Macalester College and in the Field Museum of Natural History. How to cite this article: Curry Rogers, K. et al . Sauropod dinosaur osteoderms from the Late Cretaceous of Madagascar. Nat. Commun. 2:564 doi: 10.1038/ncomms1578 (2011).